CD8+tissue-resident memory T-cell development depends on infection-matching regulatory T-cell types Immunological memory is critical for immune protection, particularly at epithelial sites, which are under constant risk of pathogen invasions. To counter invading pathogens, CD8 + memory T cells develop at the location of infection: tissue-resident memory T cells (T RM ). CD8 + T-cell responses are associated with type-1 infections and type-1 regulatory T cells (T REG ) are important for CD8 + T-cell development, however, if CD8 + T RM cells develop under other infection types and require immune type-specific T REG cells is unknown. We used three distinct lung infection models, to show that type-2 helminth infection does not establish CD8 + T RM cells. Intracellular (type-1) and extracellular (type-3) infections do and rely on the recruitment of response type-matching T REG population contributing transforming growth factor-β. Nevertheless, type-1 T REG cells remain the most important population for T RM cell development. Once established, T RM cells maintain their immune type profile. These results may have implications in the development of vaccines inducing CD8 + T RM cells. Epithelial barriers are prime portals for microbial invasion. Organ structure, such as a multilayer of epithelial cells in the skin, provides additional protection against invasion. Other organs, such as the intestine and lung require optimal exchange of nutrients, liquids, and gasses that necessitate a single epithelial cell layer. It is highly beneficial to the host to contain invading pathogens at the site of entry and swiftly clear any pathogens and their products to avoid tissue damage and systemic dissemination of infectious or toxic material. For this reason, the immune response is tailored to the identity of the invading microbe, towards intracellular (type-1), helminths (type-2), or extracellular (type-3) pathogens. Understanding how tissue immunity is established following distinct responses has conceivable therapeutic potential with the ability to modulate tissue-specific immunity, from vaccination strategies to tumour treatment. The development of immunological memory is a pillar of adaptive immunity and an efficacious way to prevent the development of disease caused by pathogen entry. Memory T lymphocytes are functionally and phenotypically classified in at least three subsets. Central memory (T CM ) and effector memory (T EM ) T cells recirculate throughout lymphoid and non-lymphoid organs respectively [1] . T EM cells actively scout for pathogens, entering and exiting organs via the circulation and lymph, while T CM cells are more quiescent and are reactivated in secondary lymphoid organs, faster than, but not dissimilarly from, naïve T cells [2] , [3] . Although these cells provide significant protection from recurrent infections due to increased antigen-specific numbers and speed of activation, they require a systemic immune reaction for triggering and may not be sufficiently efficacious against pathogen entry. Tissue-resident memory (T RM ) T cells reside in tissues, especially those at the host/environment interface. T RM cells actively survey the tissues for signs of infection, able to react rapidly and thereby swiftly eliminate infected cells without the need for a systemic immune reaction [1] . CD8 + T RM cells are characterised by the expression of different markers and transcription factors, which depend on their activation status and on the tissue type they home to [4] . Most T RM cells constitutively express CD69, which antagonises the egress receptor S1P receptor 1, thus maintaining tissue residency [5] , [6] , [7] , with organ specificity [8] . The integrins CD103 and CD49a are additional markers of tissue residency, although T RM cells negative for CD103 have been reported and CD49a may reflect activation status [9] , [10] , [11] , [12] . CD103, integrin αE pairing with β7, is mostly present on epithelial residing T RM cells, providing support for tissue homing and maintenance via epithelial cell E-cadherin binding, while potentiating cytolytic activity. Of additional importance is the absence of Killer Cell Lectin Like Receptor G1 (KLRG1), typically described as a terminal differentiation marker on effector T cells [13] , [14] . KLRG1 may compete with CD103 for the binding to E-cadherin, with its downregulation contributing to T RM cell residency [15] . A transcriptional programme, distinct from other CD8 + T-cell subsets, drives surface markers and function of T RM cells. T RM cells express low levels of Tbox protein expressed in T cells (Tbet) and Krüppel-like Factor 2 (KLF2), while Eomesodermin (Eomes) is absent [6] , [14] , [16] . Instead, T RM cells express high levels of arylhydrocarbon receptor (AhR) in gut and skin, Hobit and Blimp-1 [17] , [18] . In addition, T RM cells are maintained in a semi-activation state and distinct metabolic wiring takes place, ensuring rapid full activation when required [19] , [20] .Thus, T RM cells patrol non-lymphoid organs and perform immunosurveillance by killing infected cells and producing cytokines to recruit other immune cells to quickly eliminate the pathogen [21] , [22] . Exacerbated T-cell responses can result in tissue damage, and a balance between pathogen elimination and immunopathology needs to be maintained. Regulatory T cells (T REG ), characterised by the expression of Forkhead box protein 3 (Foxp3) transcription factor, play an important role in reducing excessive immune responses. T REG can influence the transition of effector CD8 + T cells to memory cells by limiting interleukin (Il)−2 availability, producing Il-10 and cytotoxic T-lymphocyte associate protein-4 (CTLA-4) [23] , [24] , [25] . Of importance, T REG cells can adopt a transcriptional programme in line with the type of inflammation and the CD4 + T helper (T H ) subset involved. Besides Foxp3, T REG cells can co-express the T H 1 cell (type-1) factor Tbet, the T H 2 cell (type-2) factor Gata-3, and the T H 17 cell (type-3) factor Rorγt, to take on characteristics of one of these T H cell ineages [22] , [26] , [27] , [28] . We previously showed that type-1 T REG cells, recruited via their Tbet-dependent expression of the chemokine receptor CXCR3, supply and activate transforming growth factor (TGF)β locally, thereby efficiently facilitating the generation of T RM cells [14] . However, although T RM cells were found reduced in several organs, the link between their generation and type-1 T REG cells was established in the intestine and during a type-1 immune response. This raises the question of whether the establishment of T RM cells in another organ is also dependent on type-1 T REG cells, and more importantly, whether T RM cell development during other types of infection is dependent on the corresponding type of T REG cell or remains dependent on type-1 T REG cells. Here, we show that, in the lung, type-1 T REG cells are required to establish T RM cells upon type-1 infection, while a type-2 infection does not establish a robust T RM cell population. Furthermore, type-3 infection in the same organ requires type-3 T REG cells and their provision of TGFβ for efficient T RM cell establishment. Type-1 immunity induces T RM cells in lungs In the absence of type-1 T REG , there is a reduction in CD8 + T RM cells in the intestine, lungs, and liver, due to inhibition of their generation [14] . To establish a robust infection model in the lungs, we infected Foxp3 WT mice with influenza H3N2 (X-31). A week after influenza infection, a robust influx of CD4 + and CD8 + T cells is observed (Supplementary Fig. 1a–d ). Influenza challenge results in a strongly polarised type-1 response with production of interferon (IFN)-γ and dominance of CXCR3-expressing CD4 + and CD8 + T cells, with no other polarised T-cell response observed (Fig. 1a–d ; Supplementary Fig. 1e–h ). In addition to the type-1 response of CD4 + and CD8 + T cells, predominantly type-1 T REG cells expressing CXCR3 (Fig. 1e–f ) are recruited to the site of inflammation. Fig. 1: Type-1 TREG cells are required for TRM cell generation in the lungs upon Influenza infection. Mice were infected or not intranasally with 1000 plaque-forming units (PFU) of Influenza A X-31 strain (H3N2). 10 days post-infection lungs were collected, and cells were isolated and analysed via flow cytometry for cytokine production. a Numbers of activated (CD44 + ) CD4 + T cells producing indicated cytokines ( p (Non-infected vs. Influenza H3N2) < 0.000001) and ( b ) representative flow cytometry plots ( n = 6, non-infected, n = 7 infected, N = 3). c Numbers of activated CD8 + T cells producing indicated cytokines ( p (Non-infected vs. Influenza H3N2) = 0.000013) and d representative flow cytometry plots ( n = 6, non-infected, n = 7 infected, N = 3). e , f Foxp3 WT mice ( n = 6, non-infected, n = 7 infected, N = 3) were assessed for e percentage ( p (Non-infected vs. Influenza H3N2) <0.000001), and f numbers of chemokine receptors CXCR3, ST2 (IL-33R) and CCR6 expression ( p (Non-infected vs Influenza H3N2) : CXCR3, p = 001415; ST2, p = 0.000502; CCR6, p = 0.001132), on T REG cells ( n = 6, non-infected, n = 8 infected, N = 3). g , h Mice analysed via flow cytometry for g percentages of total CD8 + T cells and h numbers of T RM cells, defined as CD69 + KLRG1 − CD8 + T cells, p ( Non - infected vs Influenza H3N2) < 0.0001 ( n = 6, N = 3). i Foxp3 WT and Foxp3 ΔTbx21 mice received CD8 CD45.1 T cells intravenously, one day prior to infection. 14 days post infection, lung cells were assessed by flow cytometry for the percentage of T RM cells (CD69 + KLRG1 - CD103+) in the transferred population (Foxp3 WT n = 17, Foxp3 ΔTbx21 n = 10, N = 4), p (Foxp3WT vs Foxp3ΔTbx21) <0.0001. Two-sided Mann–Whitney analysis was applied to compare groups. Data are presented as bars of mean ± SEM with single data points. Full size image Influenza infection results in the establishment of a substantial CD8 + T RM cell population (Fig. 1g–h ). To understand if their establishment in the lungs upon influenza infection is dependent on type-1 T REG cells we make use of our previously setup transfer model whereby CD45.1 expressing CD8 + T cells (CD8 CD45.1 ) are transferred into control Foxp3 Wt mice or Foxp3 ΔTbx21 mice that miss type-1 T REG [14] . Cells are readily recovered in the spleens, and the characteristic weight loss is observed (Supplementary Fig. 1i–k ). As previously shown in the small intestine, the absence of type-1 T REG cells reduces the establishment of CD8 + T RM cells, after CD8 CD45.1 transfer. We now extend this observation to the lungs upon influenza infection where compared to controls (Foxp3 WT ), the absence of type-1 T REG cells leads to reduced efficiency of CD8 + T RM cell development (Fig. 1i ). Type-2 immunity does not induce de novo CD8 + T RM cells in lungs Establishment of CD8 + T RM cells in the lung with similar requirements to the small intestine may still rely on the type-1 inflammation induced by an intracellular pathogen as influenza virus. We subsequently used the helminth Nippostrongylus brasiliensis , widely used as a model to elicit strong type-2 immunity in the lungs [29] . A week after infection we observe a strong activation of CD4 + T cells, CD44 hi , and a response characterised by T H 2 cells in the lungs expressing IL-4 and IL-13 (Fig. 2a, b ; Supplementary Fig. 2a, b ) [30] . However, the CD8 + T-cell compartment shows a very limited effector CD44 hi CD8 + T-cell response, without type-2 polarisation, with primarily IFN-γ produced (Fig. 2c, d ). There is an influx of T REG cells, but without a polarisation towards any specific T REG subset (Fig. 2e, f ). Although some endogenous CD8 + T RM cell accumulation is observed, the CD8 T-cell activation in the lungs is modest (Fig. 2g, h , Supplementary Fig. 2c, d ). Fig. 2: Type-2 Nippostrongylus brasiliensis infection does not yield CD8 TRM cell formation. Mice were subcutaneously infected or not with 300 stage L3 larvae of Nippostrongylus brasiliensis . 7 days post-infection lungs were collected, and cells were isolated and analysed via flow cytometry for cytokine production, and T RM cells. a Numbers of activated (CD44 + ) CD4 + T cells producing indicated cytokines, p (Non-infected vs Nippostrongylus brasiliensis ) : IFN-γ, p = 0.001749; IL-17, p = 0.002537; IL-4, p = 0.000048; IL-13, p = 0.000729, and b representative flow cytometry plots (non-infected n = 6, infected n = 9, N = 3). c Numbers of activated CD8 + T cells producing indicated cytokines and d Representative flow cytometry plots of cytokine production in CD8 + T cells (non-infected n = 6, infected n = 9, N = 3). e , f Foxp3 WT mice were assessed for e percentage and f numbers of chemokine receptors CXCR3, ST2 (IL-33R) and CCR6 expression on T REG cells, p (Non-infected vs Nippostrongylus brasiliensis ) : CXCR3, p = 0.014118; ST2, p = 0.023778; CCR6, p = 0.028885, (non-infected n = 6, infected n = 9, N = 3). g , h CD69 + KLRG1 − CD8 + T RM cell g percentage of total CD8 + T cells, p (Non-infected vs Nippostrongylus brasiliensis ) = 0.0004, and h number, p (Non-infected vs Nippostrongylus brasiliensis ) = = 0.0016, in non-infected (control) and infected mice (non-infected n = 6, infected n = 9, N = 3). i – l Foxp3 WT mice received CD8 CD45.1 T cells intravenously, one day prior to infection. 14 days post-infection, lung cells were analysed via flow cytometry for i total number of CD8 CD45.1 T cells, CD69 + KLRG1 − CD8 + T RM cell j percentage and k numbers, and l representative flow plot, within the CD8 CD45.1 T-cell population ( n = 7, N = 3). m , n Comparison of transferred CD8 CD45.1 T-cell number in the ( m ) spleen, p (Influenza vs Nippostrongylus brasiliensis ) = 0.0012, or ( n ) lungs, p (Influenza vs Nippostrongylus brasiliensis ) = 0.0002, of mice infected with Influenza and N. brasiliensis ( Influenza n = 9, N. brasiliensis n = 7, N = 3). 2-sided Mann–Whitney analysis was applied to compare the differences between groups. Data is presented as bars of mean ± SEM with single data points. Full size image CD8 CD45.1 and CD4 CD45.1 T cells transferred into Foxp3 Wt mice are recovered from the spleen, with robust numbers but without signs of activation with the majority of cells showing a naïve or T CM cell phenotype (Supplementary Fig. 2e–g ). CD8 CD45.1 T cells are few in the lungs upon infection, with CD8 + T RM cells rare and often below the detection threshold (Fig. 2i–l ). CD4 CD45.1 T cells are more numerous in the lungs upon infection, at cost of cell numbers in the spleen, with CD4 + T RM cell proportions much higher than CD8 + T RM cells (Supplementary Fig. 2g–h ). This indicated robust CD4 + T-cell recruitment to the site of N . brasiliensis infection as opposed to CD8 + T cells. Comparing influenza and N . brasiliensis , CD8 CD45.1 T cells remain abundant upon type-2 infection in the spleen, while transferred CD8 + T cells are recruited to the site of infection only after challenge with influenza (Fig. 2m, n ). Although CD8 + T RM cell generation is efficient in lung tissue, with CD8 + T cells recruited and relying on type-1 T REG cell help during a type-1 immune response, a type-2 infection, despite a robust CD4 + T-cell response (Fig. 2a, b ), does not result in de novo CD8 + T-cell recruitment, activation or polarisation, the recruitment of type-2 T REG cells, or the establishment of CD8 + T RM cells. Type-3 immunity does induce CD8 + T RM cells in lungs Besides intracellular pathogens resulting in robust CD8 + T RM cell development, we asked if extracellular pathogens, not helminths, would result in the generation of CD8 + T RM cells. Aspergillus fumigatus infection results in a robust response dominated by T H 17 cells (Fig. 3a, b ; Supplementary Fig. 3a, b ) [31] . In contrast to a type-2 infection, a type-3 challenge shows a type-1 response with increased numbers of T H 1 accompanied by a robust CD44 hi effector CD8 + T-cell response, but with few expressing IFN-γ, yet IL-17 production is observed (Fig. 3c, d ; Supplementary Fig. 3c, d ). Fig. 3: Type-3 Aspergillus fumigatus infection yields CD8 T-cell recruitment and TRM cell formation. Mice were intranasally challenged four times every 3 days with 10 6 spores of Aspergillus fumigatus . 10 days post-infection lungs were collected, and cells were isolated and analysed via flow cytometry for cytokine production, and T RM cells. a Numbers of activated (CD44 + ) CD4 + T cells producing indicated cytokines, p (Non-infected vs Aspergillus ) : IFN-γ, p = 0.005452; IL-17, p = 0.000733; IL-4, p = 0.007702; IL-13, p = 0.000005, and b representative flow cytometry plots of cytokine production in CD4 + T cells (non-infected n = 10, infected n = 12, N = 4). c Numbers of activated CD8 + T cells producing indicated cytokines, p (Non-infected vs Aspergillus ) : IFN-γ, p = 0.000951, and d representative flow cytometry plots of cytokine production in CD8 + T cells (non-infected n = 10, infected n = 14, N = 4). e , f T REG cells from Foxp3 WT mice were assessed for expression in e percentage, p (Non-infected vs Aspergillus ) : Tbet, p = 0.018008; RORγt, p = 0.001023, and f numbers, p (Non-infected vs Aspergillus ) : Tbet, p = 0.022810; RORγt, p = 0.000093, of the transcription factors Tbet, GATA-3 and RORγt in (non-infected n = 6, infected n = 7, N = 3). g , h Analysis of CD69 + KLRG1 - CD8 + T RM cell ( g ) percentage, p (Non-infected vs Aspergillus ) = 0.000017, within the total CD8 + T-cell population, and h number, p (Non-infected vs Aspergillus ) = 0.002175 in the lungs of non-infected (control) and infected mice ( n = 10, non-infected, n = 14 infected, N = 3). i Comparison of transferred CD8 CD45.1 CD69 + KLRG1 − CD8 + T RM cell numbers in the lungs upon Nippostrongylus brasiliensis (N.b.) or Aspergillus fumigatus (A.f.) infection, p (Aspergillus vs Nippostrongylus brasiliensis) =0.0012, ( n = 7, N = 3 for N.b. ; n = 6 and N = 3 for A.f). Two-sided Mann-Whitney analysis was applied to compare the differences between groups. Data is presented as bars of mean ± SEM with single data points. Full size image The influx of T REG cells shows skewing towards type-3 T REG at cost of type-1 T REG cells, with total T REG cell numbers increasing for all subsets (Fig. 3e, f ). The T REG cell response reflects the CD4 + T-cell response, which shows strong skewing towards Rorγt + CCR6 + T H 17 cells, but with increased numbers in all subsets (Supplementary Fig. 3e–g ). The proportional distribution of CD8 + T cells remains similar to uninfected, but with total numbers of type-3 CD8 + T cells increasing (Supplementary Fig. 3h–j ). Aspergillus infection increases endogenous host CD8 + T RM cell numbers in the lungs (Fig. 3g, h ). Upon adoptive transfer of CD8 CD45.1 T cells, in contrast to the type-2 infection used, newly established CD8 + T RM cells were more robustly detected upon Aspergillus challenge compared to N . brasiliensis infection (Fig. 3i ). In summary, type-1 and 3 infections result in CD8 + T RM cell formation, which is not observed for a type-2 immune response. Deletion of Rorγt in FoxP3 + cells ablates type-3 T REG cells Our results using the type-3 immunity-inducing fungi Aspergillus indicate that CD8 + T RM cells are induced during type-3 infections. This raises the question if T REG cells are required and if the type of T REG cell needs to match the infection type to efficiently establish CD8 + T RM cells after type-3 infections. In order to address this, we generated Foxp3-yfp-Cre Rorγt f/f mice (Foxp3 ΔRorγt ), in which type-3 T REG cells are efficiently removed similarly as to type-1 T REG cells in Foxp3 ΔTbx21 mice, in all tissues assayed (Fig. 4a, b ) [14] . CD4 + or CD8 + T-cell proportions or numbers, including Rorγt-expressing subsets such as T H 17 cells, or T REG subset proportions and numbers are not altered in Foxp3 ΔRorγt mice compared to controls (Fig. 4b–d ; Supplementary Fig. 4a–d ). Since type-1 T REG cells are important in CD8 + T RM cell formation [14] , we also determined proportion and numbers of type-1 T REG cells and CXCR3 expression. These are similar between Foxp3 Wt and Foxp3 ΔRorγt mice (Fig. 4b, e, f ; Supplementary Fig. 4c, e ). In agreement with the presence of similar numbers of type-1 T REG cells, the number of intraepithelial lymphocytes (IELs) and CD8 + T RM cells in the lamina propria lymphocytes (LPL), lung, and liver, which differ in Foxp3 ΔTbx21 mice [14] , were comparable between Foxp3 Wt and Foxp3 ΔRorγt mice (Fig. 4g ; Supplementary Fig. 4f–h ). Collectively, the data shows that efficient deletion of type-3 T REG cells is established without effects on other T-cell populations, as well as a noticeable effect on CD8 + T RM cells present at steady state. Fig. 4: Type-3 TREG cells are ablated in Foxp3-CreeYFP RORγtfl/fl mice. Foxp3 WT and Foxp3 ΔRORγt mice were analysed at steady-state for T REG , CD4 + , and CD8 + T cells in lung, spleen, small intestine lamina propria lymphocytes (LPL), and small intestine intraepithelial lymphocytes (IEL). a Representative flow plot of RORγt expression in LPL T REG cells in both mouse lines. b Percentage of LPL T REG cells expressing Tbet, GATA-3 or RORγt, p (Foxp3WT vs Foxp3ΔRORγt) < 0.000001, (Foxp3 WT n = 8, Foxp3 ΔRORγt n = 9, N = 3). c Percentage of RORγt expression in CD4 + and CD8 + LPL (Foxp3 WT n = 8, Foxp3 ΔRORγt n = 9, N = 3). d – f CD8 + T-cell proportions in the spleen were assessed for d naive (T N CD44 − CD62L + ), central memory (T CM , CD44 + CD62L + ) and effector memory/effector (T EM /T EFF , CD44 + CD62L − ) and e for CXCR3 expression on CD4 + , CD8 and T REG cells, with f representative flow plot ( n = 8, N = 3). g Percentage of CD69 + KLRG1 - CD103 + CD8 + T RM cell in small intestine LPL and IEL in both mouse lines (LPL Foxp3 WT n = 7, Foxp3 ΔRORγt n = 8, N = 3 ; IELs n = 6, N = 2). Two-sided Mann–Whitney analysis was applied to compare the differences between groups. Data is presented as bars of mean ± SEM with single data points. Full size image Deletion of type-3 T REG cells impacts CD8 + T RM cell formation Segmented filamentous bacteria (SFB) are known inducers of T H 17 cells [32] . However, in our hands, there was a modest induction of T H 17 cells, accompanied by T H 1 cells as well, resulting in a mixed type-1/type-3 response (Supplementary Fig. 5a, b ). In accordance, T REG cell recruitment was similar among the major three subsets (Supplementary Fig. 5c, d ). Foxp3 ΔRorγt mice mount a similar T H 1 and T H 17 cell response compared to Foxp3 Wt controls (Supplementary Fig. 5e, f ). SFB infection results in substantial CD8 + T RM cell establishment, but with reduced development in the absence of type-3 T REG cells (Fig. 5a, b ). However, the chronicity of SFB in the intestinal tract prohibits the further assessment of memory T-cell responses [32] . Fig. 5: Depletion of Type-3 TREG cells reduces TRM cell development in type-3 infections. a , b In Foxp3 WT and Foxp3 ΔRORγt mice, CD45.1 + CD8 + T cells were transferred one day prior to infection with 100 mg of segmented filamentous bacteria (SFB)-containing feces, organs were assessed for their T RM cell phenotype (CD69 + Eomes - CD103 + ) 14 days later. Small intestine LPL were collected and assessed for the T-cell phenotype of CD45.1 + CD8 + T RM cells. a Representative flow cytometry plots and b percentages of T RM cells, p (Foxp3WT vs Foxp3ΔRORγt) = 0.0357, (Foxp3 WT n = 3, Foxp3 ΔRORγt n = 5, N = 3). c , d Intranasal challenge with 1000 PFU of Influenza X-31 strain (H3N2). Lungs were collected and transferred T cells were analysed. c Representative flow cytometry plots of T RM cells within transferred T cells and d percentages of T RM cells in indicated mouse lines (Foxp3 WT n = 17, Foxp3 ΔRORγt n = 6, N = 4). e – g Mice were infected by four intranasal challenges with 10 6 spores of Aspergillus fumigatus . Lungs were collected and e total CD4 + T cells (Foxp3 WT n = 7, Foxp3 ΔRORγt n = 6, N = 3), f total T REG cells, p (Foxp3WT vs Foxp3ΔRORγt) =0.0043, and g subsets of T REG cells based on their transcription factor expression, p (Foxp3WT vs Foxp3ΔRORγt) = 0.000001, were analysed (Foxp3 WT n = 6 Foxp3 ΔRORγt n = 5, N = 3). h , i Mice were transferred with indicated condition receiving control or TGFβ1–deficient T REG cells prior to the first of four intranasal challenges with 10 6 spores of Aspergillus fumigatus . Lungs were collected and transferred CD45.1 CD8 T cells were analysed. h Representative flow cytometry plots of T RM cells within transferred CD45.1 CD8 T cells and i percentages of T RM cells in all conditions, p (Foxp3WT vs Foxp3ΔRORγt) = 0.0087, p (Foxp3ΔRORγt vs Foxp3ΔRORγt+WT Tregs) = 0.0173, p (Foxp3ΔRORγt vs Foxp3ΔRORγt+TregΔTGFβ1) = 0.0043 (Foxp3 WT ; Foxp3 ΔRORγt n = 6, N = 4; Foxp3 ΔRORγt + T REG WT n = 5, N = 2; Foxp3 ΔRORγt + T REG ΔTGFβ1 n = 5, N = 2). Multiple unpaired t test was used for g , other panels two-sided Mann-Whitney analysis was applied to compare groups. Data is presented as bars of mean ± SEM with single data points. Full size image Influenza virus causes a strong type-1 response and establishment of CD8 + T RM cells in the lung, dependent on type-1 T REG cells (Fig. 1 ). Upon infection, Foxp3 ΔRorγt and Foxp3 Wt animals showed a similarly robust development of CD8 + T RM cells (Fig. 5c, d ), in stark contrast to Foxp3 ΔTbx21 mice (Fig. 1i ), indicating primarily a dependency on type-1 T REG cells for CD8 + T RM cell development. This raised the question if Aspergillus infection, resulting in a strong type-3 response (Fig. 3 ), requires type-3 T REG cells for optimal CD8 + T RM cell development. Upon Aspergillus infection the influx of CD4 + T cells is similar between Foxp3 Wt and Foxp3 ΔRorγt animals (Fig. 5e ). However, the recruitment of T REG cells is significantly lower (Fig. 5f ), explained by the absence of type-3 T REG cells (Fig. 5g ). This is similar to our previous observations in type-1 infections in Foxp3 ΔTbx21 animals [14] . Genetic ablation of type-3 T REG cells in Foxp3 ΔRorγt animals resulted in a marked reduction of CD8 + T RM development compared with Foxp3 Wt animals (Fig. 5g, h ). Importantly, and in line with previous results obtained with type-1 pathogens (Fig. 1 ) [14] , co-transfer of control T REG cells into type-3 T REG –deficient hosts prior to a type-3 infection is able to restore CD8 + T RM cell development and numbers to the level seen in control mice, which also for type-3 responses relies on T REG cell provision of TGFβ (Fig. 5i , Supplementary Fig. 5i ). Collectively, our data suggest that there appears to exist a matching of pathogen type and T REG subset during type-1 and type-3 infections. Influenza, SFB and Aspergillus , show a dominant dependency of the equivalent T REG subset for efficient CD8 + T RM cell development. CD8 + T RM cell identity is maintained after infection Eimeria vermiformis (Ev) is a small intestinal single-cell intracellular parasite that invades small intestine epithelial cells, it is mouse-specific and self-limiting, making it an ideal tool to study T RM cell development [14] . It undergoes at least three rounds of asexual replication, each time bursting out of an infected epithelial cell to reach distal uninfected epithelial cells [33] . Its clearance depends on a type-1 inflammatory response, as we showed previously, and establishes type-1 T REG -dependent CD8 + T RM cells [14] . We tested if the establishment of CD8 + T RM cells is inhibited by the absence of type-3 T REG cells in Foxp3 ΔRorγt mice. Foxp3 ΔRorγt mice do show reduced CD8 + T RM cell development compared to Foxp3 Wt controls, although the decrease is not as marked as in the absence of type-1 T REG . (Fig. 6a, b ) [14] . Fig. 6: Type-1 and type-3 TREG cells enhance TRM cell development, the identity of which are maintained. Mice were transferred with CD45.1 + CD8 + T cells one day prior to oral gavage infection. 14 days after transplant, tissues were collected and assessed for their T RM phenotype. a , b Infection with 5000 oocysts of Eimeria vermiformis , a representative flow cytometry plots T RM cells (CD69 + Eomes - CD103 + ) and b percentages of T RM cells in both mouse lines, p (Foxp3WT vs Foxp3ΔRORγt) = 0.0020, (Foxp3 WT n = 4, Foxp3 ΔRORγt n = 10, N = 3). c , d Mice were challenged four times intranasally with 10 6 spores of Aspergillus fumigatus . Lungs were collected and transferred T cells were analysed, c representative flow cytometry plots of T RM cells and d percentages of T RM cells in both mouse lines, p (Foxp3WT vs Foxp3ΔTbet) = 0.0238 (Foxp3 WT n = 6, N = 4, Foxp3 ΔTbx21 n = 3, N = 3). e , f Mice were transferred with CD45.1 CD8 T cells prior to the first of four intranasal challenges with 10 6 spores of Aspergillus fumigatus . Lungs were collected and transferred CD45.1 CD8 + T RM cells were analysed for e IFNγ or f IL-17 production (Foxp3 WT n = 4, Foxp3 ΔRORγt n = 7, Foxp3 ΔTbx21 n = 4, N = 3). Two-sided Mann–Whitney analysis was applied to compare groups. Data is presented as bars of mean ± SEM with single data points. Full size image CD8 + T cells are strongly associated with type-1 responses. We observed IFNγ-producing CD8 + T cells also in type-2 and type-3 infections (Figs. 2c, d , 3c, d ). Hence, we next questioned if, in a strong type-3 infection model such as Aspergillus , the subsequent CD8 + T RM cell establishment that is dependent on type-3 T REG cells (Fig. 5e, f ), shows any dependency on type-1 T REG cells as is the case with Ev infection (Fig. 6a, b ). In the case of Aspergillus , the absence of either type-3 or type-1 has marked effects on the generation of CD8 + T RM cells (Figs. 5e, f , 6c, d ). Since memory T cells are maintained to offer protection against future challenges, we wished to know if CD8 + T RM cells developed under polarising conditions of type-1 or type-3 infections reflected the original skewing. We assessed the endogenous CD8 + T RM cell population after the clearance of infection. Upon influenza infection, the established CD8 + T RM cells show a predominant skewing towards the original type-1 response, with the cells mainly able to produce IFNγ (Supplementary Fig. 6a–c ). Upon an Aspergillus infection, the remaining CD8 + T RM cells are fewer and the skewing is less apparent. The recall response shows IL-17 production, in line with the initial type-3 immune response, but there is the presence of IFNγ-producing CD8 + T RM cells as well (Supplementary Fig. 6d–f ). To analyse the polarisation of newly recruited CD8 + T cells upon an Aspergillus challenge at the site of infection, we made use of our CD45.1 T-cell adoptive transfer model. The Aspergillus challenge shows a mixed type-1 and type-3 polarisation of established CD8 + T RM cells, indicating their polarisation is maintained after T RM cell development (Fig. 6e–f ). Furthermore, this model allows the assessment of the role of T REG cell types on T RM cell polarisation. Although type-1 and type-3 T REG cells enhance the establishment of T RM cells upon Aspergillus infection (Fig. 5 ), the absence of either type-1 or type-3 T REG cells does not alter the polarisation toward the production of IFNγ or IL-17 (Fig. 6e, f ). Our data suggest that CD8 + T RM cell formation occurs predominantly during type-1 immune responses, largely depending on type-1 T REG cell recruitment and action. Type-3 infections do give rise to CD8 + T RM cells as well, but these are more modest in numbers. Although there is preferential recruitment of infection-type-matching T REG cells, there is redundancy between T REG populations, especially when polarisation is less dominant. After establishment, CD8 + T RM cells maintain their original profile, determined by the infection type, after pathogen clearance. Non-lymphoid tissue immunity is important to guard against reinfection, local containment of invaders and to reduce the chance of systemic dissemination [34] . This is established after primary infection and is of great interest for vaccine strategies. T REG cells are a critical component in the management of immune responses, maintaining self-tolerance and homoeostasis. Different populations of T REG cells exist and co-localise with the corresponding CD4 + Th cell subsets, with similar transcriptional programmes and associated expression of chemokine receptors [27] , [35] , [36] . Our previous data showed the requirement of type-1 T REG cell recruitment to the site of inflammation to release and make available TGFβ, thereby facilitating CD8 + T RM cell development. The work focussed on an intestinal intracellular parasite infection, Eimeria vermiformis , invoking a type-1 dominated response with CD8 + T RM cell development dependent on type-1, Tbet- and CXCR3-expressing, T REG cells [14] . Mirroring of transcription programmes and chemokine receptor expression raised the question that particular T REG subsets may control immune responses within the context of the pathogen encountered. This suggests that the development of CD8 + T RM cells may require a match between type of infection and T REG subset to be recruited [22] . Localised infections result in strong CD8 + T RM cell development, require inflammation-mediated lymphocyte trafficking and the cognate antigen to be present in the local microenvironment [14] , [34] , [37] , [38] . Our results are obtained using three distinct infection models in the lungs. In each of the models, CD4 + T cells are recruited to the site of inflammation, and each type of infection is dominated by the corresponding T H cell subset, in numbers and proportions; Influenza by T H 1 cells (IFNγ), N. brasiliensis by T H 2 cells (IL-4, IL-13), and A. fumigatus by T H 17 cells (IL-17). A potential limitation of our analysis is that we did not in vivo label the studied cells, a method used to identify circulating cells. However, this method has some disadvantages as it does not address migration properties and, in a highly vascular organ such as the lungs, the inflammatory context might result in tissue permeability and affect the results [39] . We tested the role of type-3 T REG cells in the establishment of CD8 + T RM cells after a type-3 infection by genetically removing them using Foxp3 ΔRorγt animals. We successfully used this approach with Foxp3 ΔTbx21 animals [14] . In Foxp3 ΔRorγt animals, the total number of T REG cells, including type-1 T REG cells that contribute to CD8 + T RM cell development, T H 17 cells, and CD8 + T cells expressing Rorγt were not altered. This confirms that the Foxp3-Cre-driven deletion is T REG -specific and attests to the careful genotyping of mice used. Conform our previous results in the small intestine [14] , predominantly type-1 T REG cells are recruited upon a viral infection in the lung, which are required to enhance the establishment of CD8 + T RM cells. CD8 T cells are also recruited to the site of the influenza infection and are nearly exclusively IFNγ-producers. Although we observe a robust T H 2 cell response upon N. brasiliensis infection, and although more T REG cells are recruited, we did not see a predominance of type-2 T REG cells at the site of infection. In addition, CD8 + T cells are marginally recruited to, and activated at, the site of infection, although the presence of more endogenous CD8 + T RM cells was observed. It is not clear if these cells are an expansion of the local CD8 + T RM cell population responding to a local inflammation or if these are pathogen-specific. However, using CD45.1 adoptive transfers, it is clear that few naïve CD8 + T cells are recruited to the site of infection, while CD4 + T cells are. The cytokine expression profile of CD8 + T cells did not differ from non-infected controls, and the characteristic type-2 cytokines IL-4 and IL-13 were not detected. CD8 + T cells are not associated with type-2 or anti-helminth responses [40] . There are suggestions that helminths may themselves reduce the CD8 + T-cell response [41] . Therefore, our results may be applicable to helminth-induced type-2 responses but not represent allergic responses. Type-3-dominated infections, represented by A. fumigatus and SFB, do result in preferential recruitment of type-3 T REG cells as well as the recruitment of CD8 + T cells. However, and in contrast to CD4 + T cells, the CD8 + T cells recruited are less numerous compared to influenza. IL-17-producing CD8 + T cells are present after type-3 infection, but constitute a small population. CD8 + T RM cell development does take place, but is not as efficient as observed during a type-1 response. In contrast to Foxp3 ΔTbx21 animals in which we observe a marked decrease in CD8 + T RM cells under steady-state conditions without known infection, Foxp3 ΔRorγt animals have numbers of CD8 + T RM cells comparable to controls. This indicates that type-3 T REG cell recruitment does not make a critical contribution to the overall development of CD8 + T RM cells. Upon infection with A. fumigatus or SFBs, however, the absence of type-3 T REG cells makes CD8 + T RM cell development less efficient. We confirm that the development of CD8 + T RM cells during a type-1 infection, such as influenza, does not depend on type-3 T REG cells but on type-1 T REG cell recruitment exclusively. Less polarised responses or non-type-1 dominated infections are less dependent on specific T REG subset recruitment to facilitate CD8 + T RM cell development. This is in agreement with the T cells detected during the A. fumigatus or SFB infection showing a type-1 and type-3 identity, hence relying on type-1 and type-3 T REG cell recruitment for CD8 + T RM cell establishment. Infections are often a mixed response with type-1 responses playing an important role in most [42] . This may reflect the involvement of CD8 + T cells, which show an overwhelming type-1 dominated response. In accordance, the development of CD8 + T RM cells during type-3 responses is not exclusively dependent on type-3 T REG cell recruitment, but also on type-1 T REG cells. However, the polarisation of CD8 + T RM cells is determined by the infection and not by the recruitment of type-1 or type-3 T REG cells. In the context of any invader, the establishment of a tissue-resident T-cell memory pool will be an advantage to locally contain the infection, independent of antigen specificity [43] . The functional relevance of mismatched CD8 + T RM cells during a reinfection is speculative but type-3 responses are flexible and can be converted to give rise to type-1 cells [44] . Although largely observed on CD4 + T cells, a mixed type-1/-3 response can be beneficial to reduce pathogen load and pathology in subsequent infections [45] , [46] , [47] , [48] , [49] . In addition, tissue repair can be enhanced by type-2 responses and type-3 CD8 + T RM cells have been reported in the context of signals from injury and exposure to inflammatory mediators to release type-2 cytokines [50] . The physiological and clinical relevance of this mixed response, especially for CD8 + T RM cells, is currently not clear but a subject for future investigation. In summary, we extend previous work that T REG cells, critical in preventing autoimmunity and immunopathology, have an important role in efficiently generating tissue-resident memory T cells from effector or memory precursors. We show that type-2 helminth infections are unlikely to result in robust de novo CD8 + T RM cell formation. Type-3 infections result in CD8 + T RM cell development, but less robust than type-1 infections. Type-1 T REG cell recruitment is required for CD8 + T RM cell development during type-1 infections, although type-3 T REG cells may assist in less type-1 dominated responses, resulting in a predominantly IFNγ–producing CD8 + T RM cell population. During type-3 infection, both type-1 and -3 T REG cells play an important role, resulting in the establishment of a CD8 + T RM cell population containing a mix of IFNγ- and IL-17-producing cells. Excluding helminths, independently of the type of pathogen encountered, CD8 + T RM cells are generated, offering enhanced protection against future challenges. Mice C57BL/6 J CD45.1 mice were purchased from Charles River, France. Tbx21 fl/fl (Tbx21 tm2Srnr ) were kindly provided by Dr. Steven Reiner [51] , Foxp3eYFP-Cre (Foxp3 tm4(YFP/icre)Ayr ) was kindly provided by Dr. Alexander Rudensky [52] , Rosa26-tdRFP was kindly provided by Dr. Hans Jörg Fehling [53] . RORγt fl/fl mice were obtained on Jackson Laboratories, Foxp3eYFP-Cre TGFβ1 -/- mice were kindly provided by Dr. Julien Marie [14] . Mice were bred at the Instituto de Medicina Molecular, Lisbon, Portugal. Male and female mice, aged and sex-matched, at 12–25 weeks of age were used. Animals were housed in IVC cages with temperature-controlled conditions under a 12-h light/dark cycle with free access to drinking water and food. All mice were kept in specific pathogen-free conditions. All mice in the Foxp3eYFP-Cre Rosa26-tdRFP lines were stringently genotyped by PCR and those in which a knockout allele was detected were discarded (~20%). In addition, mice were counter-screened for inappropriate expression of RFP in relation to eYFP (~10% discarded). All animal experimentation complied with regulations and guidelines of, and was approved by, the Direção-Geral de Alimentação e Veterinária Portugal and the local ethical review committee (Orbea). Cell isolation ntestine was flushed with PBS to remove contents and opened longitudinally. After cutting into 1 cm pieces, it was incubated in PBS containing 20 mM Hepes, 100 U/ml penicillin, 100 µg/ml streptomycin, 1 mM Pyruvate, 10% FCS, 100 μg/ml polymyxin B and 10 mM EDTA for 30 min at 37 °C while shaking to release IELs. IEL single-cell suspensions were further purified using 37.5% isotonic Percoll. To isolate LPLs, intestinal tissue was then digested in IMDM medium containing 0.5 mg/ml of Collagenase D (Roche) and 0.2 mg/ml of DNaseI (Roche) for 25 min at 37 °C while shaking. Lungs were perfused with 20 mL of PBS before being shredded in small pieces with scissors and digested in IMDM medium containing 5% FBS and 0.5 mg/ml Collagenase D, 37 °C during 30 min while shaking. The cell suspension containing the lymphocytes was passed through a 50 μm cell strainer, incubated for 2 min in ACK solution, and lymphocytes were obtained after a 6-min wash with PBS at 500 g centrifugation. Adoptive cell transfers CD8α + T cells and/or CD25 + cells (T REG cells) were purified from a single-cell suspension of spleen and lymph nodes. Briefly, cells were labelled with anti-CD8a-APC or anti-CD25-APC antibodies and selected with anti-APC MACS microbeads, according to the manufacturer’s instructions. After counting, purity was determined by flow cytometry, and cell numbers were adjusted. To ensure a wide TCR diversity in the population transferred a minimum of 2 × 10 6 CD8 + T cells were used. Some of the recipient mice received in addition 0.6–1 × 10 6 T REG cells. Infection was performed one day after cell transfer (day 0). Influenza X-31 preparation and infection Reverse genetics A/X-31 (PR8-HK4 and 6) were used as model viruses. Reverse genetics derived chimeric PR8 containing the segment 4 from A/Hong Kong/1/1968, seg4-HK68 (PR8-HK4), or the segment 6 (PR8-HK6) were produced as previously described [54] , [55] , [56] . pDual plasmids were a kind gift from Dr. Ron Fouchier (Erasmus MC, Netherlands). PR8 NA-E229A [57] was generated by reverse genetics after site-directed mutagenesis of pDual::segment 6. All viruses were amplified in embryonated chicken eggs and titrated using plaque assay as previously described [58] , [59] . A viral load of 1000 PFU was administered in 30 μL PBS intranasally to mice. Mouse weight was monitored daily during the experiment to certify welfare, with mice going lower than 25% initial weight being sacrificed. Eimeria vermiformis infection Animals were infected with Eimeria vermiformis (Ev) as previously described in detail [33] . Briefly, oocysts were washed three times with deionized water, floated in sodium hypochloride and counted using a Fuchs-Rosenthal chamber. Mice received 5000 oocysts of E. vermiformis by oral gavage in 100 μl of water. N. brasiliensis infection N. brasiliensis worms were propagated as previously described [30] . Infective L3 larvae were kindly provided by Brian Chan at Dr Judith E Allen’s laboratory. Briefly, the larvae were obtained by cutting the filter paper in which they were provided around the borders (~0.5 cm), emerging it around gauze in a Falcon tube with 40 mL of PBS at 37 °C for 10 min (Baermann’s method). After this, larvae were allowed to pool down by gravity for 10 min, with the bottom 10–15 mL containing them being transferred to a 15 mL tube. The larvae were then purified by performing three washes at 168 g with minimum break. Mice were then injected with 300 L3s subcutaneously. A. fumigatus preparation and infection Fungal isolate A. fumigatus strain Af293 was purchased from the Fungal Genetics Stock Center (Kansas City, MO, United States). The fungal strain was cultivated on T-flasks containing sabouraud dextrose agar (SDA). Cultures were incubated in the dark, for 3–4 days, at 37 °C. Asexual spores (conidia) were harvested using glass beads and a saline solution B (0.85% NaCl, 0.1% Tween-20), washed twice with a saline solution A (0.85% NaCl), and collected after passing through three layers of miracloth filter. The harvested conidia were resuspended in a phosphate-buffered saline solution (0.01 M phosphate buffer, 0.0027 M potassium chloride, 0.137 M sodium chloride, pH 7.4), and kept at 4 °C until mice infection (same day). Prior to infection, conidia were counted with a hemacytometer and subsequently resuspended to a concentration of 3.3 × 10 7 conidia/mL −1 , 30 µL were used for mice infection (106 conidia). Mice were submitted to 4 intranasal challenges with 10 6 conidia every 3 days over 2 weeks. SFB fecal transplant SFB-containing feces were kindly provided by Dr. Gérard Eberl at Pasteur Institute, Paris. Fecal pellets were collected and kept at −20 °C to maintain integral microbiota. On the day of the fecal transplant, feces were defrosted, mashed, and suspended in filtered tap water at a concentration of 100 mg/mL. Mice then received a fecal transplant of 200 μL of this suspension by oral gavage. 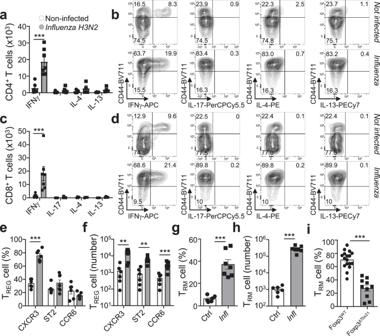Fig. 1: Type-1 TREG cells are required for TRM cell generation in the lungs upon Influenza infection. Mice were infected or not intranasally with 1000 plaque-forming units (PFU) of Influenza A X-31 strain (H3N2). 10 days post-infection lungs were collected, and cells were isolated and analysed via flow cytometry for cytokine production.aNumbers of activated (CD44+) CD4+T cells producing indicated cytokines (p(Non-infected vs. Influenza H3N2)< 0.000001) and (b) representative flow cytometry plots (n= 6, non-infected,n= 7 infected,N= 3).cNumbers of activated CD8+T cells producing indicated cytokines (p(Non-infected vs. Influenza H3N2)= 0.000013) anddrepresentative flow cytometry plots (n= 6, non-infected,n= 7 infected,N= 3).e,fFoxp3WTmice (n= 6, non-infected,n= 7 infected,N= 3) were assessed forepercentage (p(Non-infected vs. Influenza H3N2)<0.000001), andfnumbers of chemokine receptors CXCR3, ST2 (IL-33R) and CCR6 expression (p(Non-infected vs Influenza H3N2): CXCR3,p= 001415; ST2,p= 0.000502; CCR6,p= 0.001132), on TREGcells (n= 6, non-infected,n= 8 infected,N= 3).g,hMice analysed via flow cytometry forgpercentages of total CD8+T cells andhnumbers of TRMcells, defined as CD69+KLRG1−CD8+T cells,p(Non-infected vs Influenza H3N2)< 0.0001 (n= 6,N= 3).iFoxp3WTand Foxp3ΔTbx21mice received CD8CD45.1T cells intravenously, one day prior to infection. 14 days post infection, lung cells were assessed by flow cytometry for the percentage of TRMcells (CD69+KLRG1-CD103+) in the transferred population (Foxp3WTn= 17, Foxp3ΔTbx21n= 10,N= 4),p(Foxp3WT vs Foxp3ΔTbx21)<0.0001. Two-sided Mann–Whitney analysis was applied to compare groups. Data are presented as bars of mean ± SEM with single data points. Flow cytometry Single-cell suspensions from spleen, intestine, and lung were prepared and stained with antibodies (Supplementary Table 1 ), according to the agreed standards [60] . For intracellular cytokine staining, cells were pre-stimulated with PDBU (Phorbol 12,13-dibutyrate) (0.5 µg/mL) and ionomycin (0.5 μg/mL), in the presence of Brefeldin A (2 μg/mL) (all from Sigma) for 2 h at 37 °C. Samples were run on a Fortessa X20 cytometer (BD Biosciences) and analysed with FlowJo X software (TreeStar) (Supplementary Fig. 7 ). Statistical analysis In the present work, statistical analyses were performed using GraphPad Prism Software (GraphPad Prism version 9 for Windows, GraphPad Software, San Diego, California USA), details described in each figure legend where applicable. N denotes the number of independent biological repeats and n the total number of samples (mice). Error bars represent S.E.M. 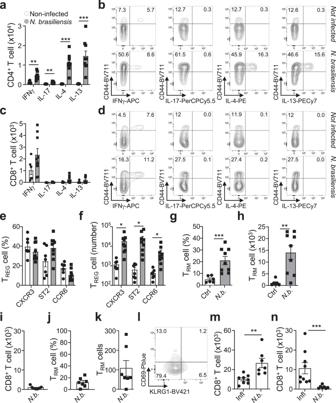Fig. 2: Type-2 Nippostrongylus brasiliensis infection does not yield CD8 TRM cell formation. Mice were subcutaneously infected or not with 300 stage L3 larvae ofNippostrongylus brasiliensis. 7 days post-infection lungs were collected, and cells were isolated and analysed via flow cytometry for cytokine production, and TRMcells.aNumbers of activated (CD44+) CD4+T cells producing indicated cytokines,p(Non-infected vsNippostrongylus brasiliensis): IFN-γ,p= 0.001749; IL-17,p= 0.002537; IL-4,p= 0.000048; IL-13,p= 0.000729, andbrepresentative flow cytometry plots (non-infectedn= 6, infectedn= 9,N= 3).cNumbers of activated CD8+T cells producing indicated cytokines anddRepresentative flow cytometry plots of cytokine production in CD8+T cells (non-infectedn= 6, infectedn= 9,N= 3).e,fFoxp3WTmice were assessed forepercentage andfnumbers of chemokine receptors CXCR3, ST2 (IL-33R) and CCR6 expression on TREGcells,p(Non-infected vsNippostrongylus brasiliensis): CXCR3,p= 0.014118; ST2,p= 0.023778; CCR6,p= 0.028885, (non-infectedn= 6, infectedn= 9,N= 3).g,hCD69+KLRG1−CD8+TRMcellgpercentage of total CD8+T cells,p(Non-infected vsNippostrongylus brasiliensis)= 0.0004, andhnumber,p(Non-infected vsNippostrongylus brasiliensis)= = 0.0016, in non-infected (control) and infected mice (non-infectedn= 6, infectedn= 9,N= 3).i–lFoxp3WTmice received CD8CD45.1T cells intravenously, one day prior to infection. 14 days post-infection, lung cells were analysed via flow cytometry foritotal number of CD8CD45.1T cells, CD69+KLRG1−CD8+TRMcelljpercentage andknumbers, andlrepresentative flow plot, within the CD8CD45.1T-cell population (n= 7,N= 3).m,nComparison of transferred CD8CD45.1T-cell number in the (m) spleen,p(Influenza vsNippostrongylus brasiliensis)= 0.0012, or (n) lungs, p(Influenza vsNippostrongylus brasiliensis)= 0.0002, of mice infected withInfluenzaandN. brasiliensis(Influenzan= 9,N. brasiliensisn= 7,N= 3). 2-sided Mann–Whitney analysis was applied to compare the differences between groups. Data is presented as bars of mean ± SEM with single data points. Mann–Whitney analysis was applied to compare ranks between two groups with a p value of 0.05. * P < 0.05, ** P < 0.01, *** P < 0.001. 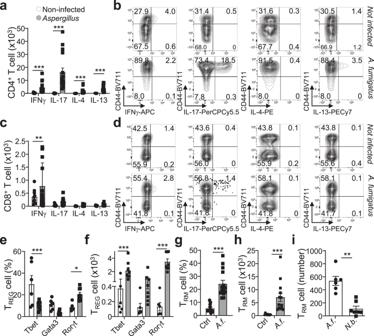Fig. 3: Type-3 Aspergillus fumigatus infection yields CD8 T-cell recruitment and TRM cell formation. Mice were intranasally challenged four times every 3 days with 106spores ofAspergillus fumigatus. 10 days post-infection lungs were collected, and cells were isolated and analysed via flow cytometry for cytokine production, and TRMcells.aNumbers of activated (CD44+) CD4+T cells producing indicated cytokines,p(Non-infected vsAspergillus): IFN-γ,p= 0.005452; IL-17,p= 0.000733; IL-4,p= 0.007702; IL-13,p= 0.000005, andbrepresentative flow cytometry plots of cytokine production in CD4+T cells (non-infectedn= 10, infectedn= 12,N= 4).cNumbers of activated CD8+T cells producing indicated cytokines,p(Non-infected vsAspergillus): IFN-γ,p= 0.000951, anddrepresentative flow cytometry plots of cytokine production in CD8+T cells (non-infectedn= 10, infectedn= 14,N= 4).e,fTREGcells from Foxp3WTmice were assessed for expression inepercentage,p(Non-infected vsAspergillus): Tbet,p= 0.018008; RORγt,p= 0.001023, andfnumbers,p(Non-infected vsAspergillus): Tbet,p= 0.022810; RORγt,p= 0.000093, of the transcription factors Tbet, GATA-3 and RORγt in (non-infectedn= 6, infectedn= 7,N= 3).g,hAnalysis of CD69+KLRG1-CD8+TRMcell (g) percentage,p(Non-infected vsAspergillus)= 0.000017, within the total CD8+T-cell population, andhnumber,p(Non-infected vsAspergillus)= 0.002175 in the lungs of non-infected (control) and infected mice (n= 10, non-infected,n= 14 infected,N= 3).iComparison of transferred CD8CD45.1CD69+KLRG1−CD8+TRMcell numbers in the lungs uponNippostrongylus brasiliensis(N.b.) orAspergillus fumigatus(A.f.) infection,p(Aspergillus vs Nippostrongylus brasiliensis)=0.0012, (n= 7,N= 3 for N.b.;n= 6 andN= 3 for A.f). Two-sided Mann-Whitney analysis was applied to compare the differences between groups. Data is presented as bars of mean ± SEM with single data points. 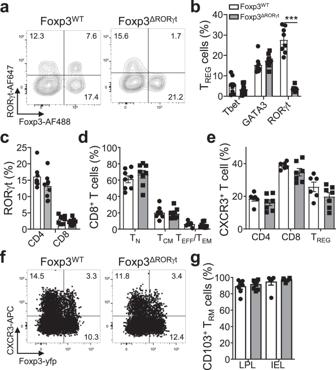Fig. 4: Type-3 TREG cells are ablated in Foxp3-CreeYFP RORγtfl/fl mice. Foxp3WTand Foxp3ΔRORγtmice were analysed at steady-state for TREG, CD4+, and CD8+T cells in lung, spleen, small intestine lamina propria lymphocytes (LPL), and small intestine intraepithelial lymphocytes (IEL).aRepresentative flow plot of RORγt expression in LPL TREGcells in both mouse lines.bPercentage of LPL TREGcells expressing Tbet, GATA-3 or RORγt, p(Foxp3WT vs Foxp3ΔRORγt)< 0.000001, (Foxp3WTn= 8, Foxp3ΔRORγtn= 9,N= 3).cPercentage of RORγt expression in CD4+and CD8+LPL (Foxp3WTn= 8, Foxp3ΔRORγtn= 9,N= 3).d–fCD8+T-cell proportions in the spleen were assessed fordnaive (TNCD44−CD62L+), central memory (TCM, CD44+CD62L+) and effector memory/effector (TEM/TEFF, CD44+CD62L−) andefor CXCR3 expression on CD4+, CD8 and TREGcells, withfrepresentative flow plot (n= 8,N= 3).gPercentage of CD69+KLRG1-CD103+CD8+TRMcell in small intestine LPL and IEL in both mouse lines (LPL Foxp3WTn= 7, Foxp3ΔRORγtn= 8,N= 3;IELsn= 6,N= 2). Two-sided Mann–Whitney analysis was applied to compare the differences between groups. Data is presented as bars of mean ± SEM with single data points. 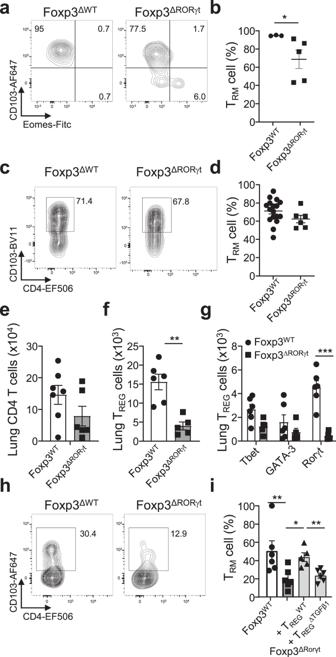Fig. 5: Depletion of Type-3 TREG cells reduces TRM cell development in type-3 infections. a,bIn Foxp3WTand Foxp3ΔRORγtmice, CD45.1+CD8+T cells were transferred one day prior to infection with 100 mg of segmented filamentous bacteria (SFB)-containing feces, organs were assessed for their TRMcell phenotype (CD69+Eomes-CD103+) 14 days later. Small intestine LPL were collected and assessed for the T-cell phenotype of CD45.1+CD8+TRMcells.aRepresentative flow cytometry plots andbpercentages of TRMcells,p(Foxp3WT vs Foxp3ΔRORγt)= 0.0357, (Foxp3WTn= 3, Foxp3ΔRORγtn= 5,N= 3).c,dIntranasal challenge with 1000 PFU of Influenza X-31 strain (H3N2). Lungs were collected and transferred T cells were analysed.cRepresentative flow cytometry plots of TRMcells within transferred T cells anddpercentages of TRMcells in indicated mouse lines (Foxp3WTn= 17, Foxp3ΔRORγtn= 6,N= 4).e–gMice were infected by four intranasal challenges with 106spores ofAspergillus fumigatus. Lungs were collected andetotal CD4+T cells (Foxp3WTn= 7, Foxp3ΔRORγtn= 6,N= 3),ftotal TREGcells,p(Foxp3WT vs Foxp3ΔRORγt)=0.0043, andgsubsets of TREGcells based on their transcription factor expression,p(Foxp3WT vs Foxp3ΔRORγt)= 0.000001, were analysed (Foxp3WTn= 6 Foxp3ΔRORγtn= 5,N= 3).h,iMice were transferred with indicated condition receiving control or TGFβ1–deficient TREGcells prior to the first of four intranasal challenges with 106spores ofAspergillus fumigatus. Lungs were collected and transferred CD45.1 CD8 T cells were analysed.hRepresentative flow cytometry plots of TRMcells within transferred CD45.1 CD8 T cells andipercentages of TRMcells in all conditions,p(Foxp3WT vs Foxp3ΔRORγt)= 0.0087,p(Foxp3ΔRORγt vs Foxp3ΔRORγt+WT Tregs)= 0.0173,p(Foxp3ΔRORγt vs Foxp3ΔRORγt+TregΔTGFβ1)= 0.0043 (Foxp3WT; Foxp3ΔRORγtn= 6,N= 4; Foxp3ΔRORγt+ TREGWTn= 5,N= 2; Foxp3ΔRORγt+ TREGΔTGFβ1n= 5,N= 2). Multiple unpairedttest was used forg, other panels two-sided Mann-Whitney analysis was applied to compare groups. Data is presented as bars of mean ± SEM with single data points. 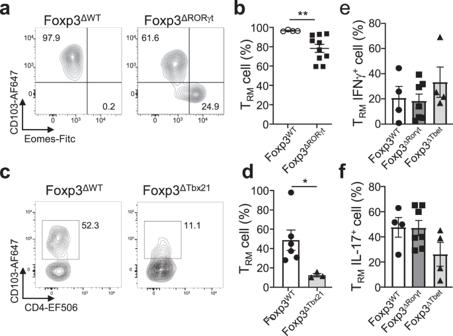Fig. 6: Type-1 and type-3 TREG cells enhance TRM cell development, the identity of which are maintained. Mice were transferred with CD45.1+CD8+T cells one day prior to oral gavage infection. 14 days after transplant, tissues were collected and assessed for their TRMphenotype.a,bInfection with 5000 oocysts ofEimeria vermiformis,arepresentative flow cytometry plots TRMcells (CD69+Eomes-CD103+) andbpercentages of TRMcells in both mouse lines,p(Foxp3WT vs Foxp3ΔRORγt)= 0.0020, (Foxp3WTn= 4, Foxp3ΔRORγtn= 10,N= 3).c,dMice were challenged four times intranasally with 106spores ofAspergillus fumigatus. Lungs were collected and transferred T cells were analysed,crepresentative flow cytometry plots of TRMcells anddpercentages of TRMcells in both mouse lines,p(Foxp3WT vs Foxp3ΔTbet)= 0.0238 (Foxp3WTn= 6,N= 4, Foxp3ΔTbx21n= 3,N= 3).e,fMice were transferred with CD45.1 CD8 T cells prior to the first of four intranasal challenges with 106spores ofAspergillus fumigatus. Lungs were collected and transferred CD45.1 CD8+TRMcells were analysed foreIFNγ orfIL-17 production (Foxp3WTn= 4, Foxp3ΔRORγtn= 7, Foxp3ΔTbx21n= 4,N= 3). Two-sided Mann–Whitney analysis was applied to compare groups. Data is presented as bars of mean ± SEM with single data points. Reporting summary Further information on research design is available in the Nature Portfolio Reporting Summary linked to this article.